Highly stable Pt monolayer on PdAu nanoparticle electrocatalysts for the oxygen reduction reaction Stability is one of the main requirements for commercializing fuel cell electrocatalysts for automotive applications. Platinum is the best-known catalyst for oxygen reduction in cathodes, but it undergoes dissolution during potential changes while driving electric vehicles, thus hampering commercial adoption. Here we report a new class of highly stable, active electrocatalysts comprising platinum monolayers on palladium–gold alloy nanoparticles. In fuel-cell tests, this electrocatalyst with its ultra-low platinum content showed minimal degradation in activity over 100,000 cycles between potentials 0.6 and 1.0 V. Under more severe conditions with a potential range of 0.6–1.4 V, again we registered no marked losses in platinum and gold despite the dissolution of palladium. These data coupled with theoretical analyses demonstrated that adding a small amount of gold to palladium and forming highly uniform nanoparticle cores make the platinum monolayer electrocatalyst significantly tolerant and very promising for the automotive application of fuel cells. One critical problem facing the proton electrolyte membrane fuel cells (PEMFCs) is the deterioration of activity during operating conditions, mainly caused by the dissolution and loss of platinum (Pt) nanoparticles at the cathode [1] , [2] , [3] , [4] , [5] . The durability of existing Pt catalysts is unsatisfactory for realizing the commercialization of PEMFCs for automotive applications. Recently, we reported on Pt monolayer shell on palladium (Pd) core nanoparticle electrocatalysts that derive stability from the protection of the shell by the core [6] . In fuel-cell tests, such an ultra-low Pt-content electrocatalyst endured 100,000 cycles at potentials between 0.7 and 0.9 V, during which no considerable loss of Pt was observed, whereas Pd underwent considerable dissolution from the cores, resulting in hollow structures. Not only did the Pd core efficiently confer stability on the Pt monolayer shell, it also enhanced its oxygen reduction reaction (ORR) activity by inducing a slight contraction in the Pt bonds that downshifts the d -band centre, thereby decreasing the reactivity of Pt [7] , [8] . This alleviates two impeding effects for ORR activity, that is, the interaction strength between Pt and ORR surface intermediates and the bonding of OH and O to Pt [9] , [10] . Here we describe our advance that we could further improve the stability of the Pt monolayer electrocatalyst by using a new, highly uniform Pd 9 Au 1 alloy core while retaining the activity of the ORR as high as that of the Pt ML /Pd/C electrocatalyst. This electrocatalyst with its ultra-low Pt content showed minimal degradation in activity (only 8%) over 100,000 cycles between potentials 0.6 and 1.0 V; this is a significant improvement compared with the Pt ML /Pd/C electrocatalyst that declined to 37% after 100,000 cycles [6] . Furthermore, under more severe test conditions involving a potential range of 0.6–1.4 V, again we registered no marked losses in Pt and Au. New mechanisms that rationalize the enhanced stability of this electrocatalyst are formulated based on the theoretical analyses and the experimental data. Considering its fuel-cell performance, particularly activity and stability, the Pt ML /Pd 9 Au 1 /C electrocatalyst appears to be a promising candidate to facilitate the automotive applications of fuel cells. 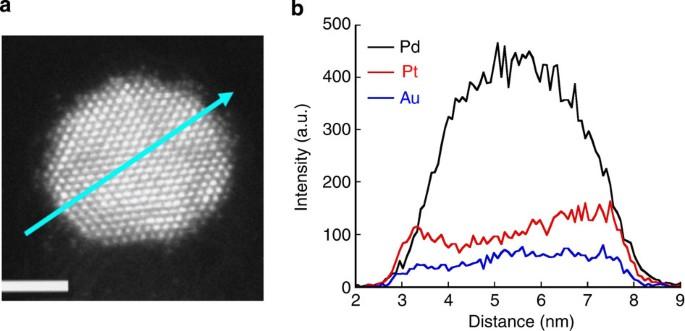Figure 1: Microscopic and compositional observations of a single Pt monolayer on a Pd9Au1nanoparticle electrocatalyst. (a) HAADF/STEM image of carbon-supported PtML/Pd9Au1nanoparticle. Bar size, 2 nm. (b) Distribution of components in the PtML/Pd9Au1nanoparticle obtained by the line-scan analysis using EDS/STEM (along the blue arrow ina). Structure of Pt ML /PdAu/C electrocatalyst Figure 1a shows a high-angle annular dark field (HAADF)/scanning transmission electron microscopy (STEM) image of a carbon-supported Pt ML /Pd 9 Au 1 nanoparticle, and a line-profile analysis using STEM/energy-dispersive spectroscopy (EDS), revealing the distribution of the Pt, Pd and Au components in the nanoparticle ( Fig. 1b ). The length of this nanoparticle is 5.4 nm as designated by the line in the figure. The profile analysis indicates that Au atoms are distributed uniformly over the Pd. The intensity of the Pt component also is continuously distributed over the nanoparticle with one intriguing feature, viz ., its concentration is slightly higher at the rims of the nanoparticle, demonstrating the formation of a core(PdAu)–shell(Pt) structure. We obtained similar EDS profiles from numerous individual nanoparticles. The mean diameter of the nanoparticles was 3.8 nm (the histograms of the particle size distribution are depicted in Supplementary Fig. S1 ). Supplementary Figure S2 illustrates the synchrotron X-ray diffraction pattern measured from the Pt ML /Pd 9 Au 1 /C nanoparticles. Therein, the two pronounced reflection peaks at 2 θ =28.283° and 32.726° are considered to correspond to the Pd(111) and Pd(200) reflections, respectively; the peaks are slightly shifted to lower angles compared with those for pure Pd metal (2 θ =28.382° and 32.889° for (111) and (200) planes, respectively) due to the formation of the PdAu solid–solution alloy nanoparticles (Pd and Au are known to form a solid–solution alloy as the bulk [11] ). No separate peaks for Pt and Au were observed, indicating that there are no large three-dimensional clusters (that is, the order of a few nanometres) of the Pt and Au single phases. Figure 1: Microscopic and compositional observations of a single Pt monolayer on a Pd 9 Au 1 nanoparticle electrocatalyst. ( a ) HAADF/STEM image of carbon-supported Pt ML /Pd 9 Au 1 nanoparticle. Bar size, 2 nm. ( b ) Distribution of components in the Pt ML /Pd 9 Au 1 nanoparticle obtained by the line-scan analysis using EDS/STEM (along the blue arrow in a ). 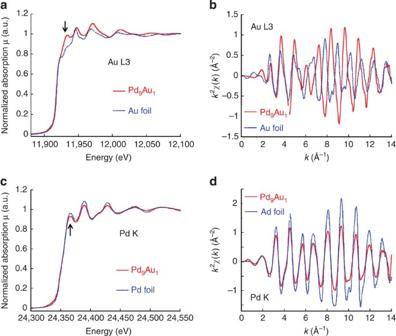Figure 2:In situX-ray absorption studies. (a,b) XANES and EXAFSk-space spectra (k2-weighted) from Au L3, and (c,d) from Pd K edges from the Pd9Au1nanoparticles measured in 1 M HClO4at a potential of 0.41 V (red lines), together with those from reference foils (blue lines). Full size image Figure 2 depicts the in situ X-ray absorption spectroscopy (XAS) of the Au L3 and Pd K edges from the Pd 9 Au 1 nanoparticles (without the Pt monolayers) in 1 M HClO 4 at a potential of 0.41 V, together with those from their respective reference foils. There is a prominent difference between Au from the Pd 9 Au 1 nanoparticles and the Au foil, both in the X-ray absorption near-edge structure (XANES) region and in the extended X-ray absorption fine structure (EXAFS) region ( k -space), respectively, in Fig. 2a,b . We note that the XANES of Au from the Pd 9 Au 1 nanoparticles also differs from those observed by others in gold (Au) oxides [12] , [13] . We attribute these dissimilarities to changes in their electronic states due to the interactions with Pd atoms. In the k -space ( Fig. 2b ), the phase in oscillation of Au from the Pd 9 Au 1 nanoparticles is shifted markedly from that apparent in the Au foil, indicating that the atomic structure significantly differs from that of an Au bulk. The XANES of Pd from Pd 9 Au 1 nanoparticles ( Fig. 2c ) is very distinguishable from that from a foil, pointing to electronic interference from Au atoms. On the other hand, the phase in oscillation in the k -space ( Fig. 2d ) is not particularly unlike from those from a Pd foil, although the amplitude of the former is slightly smaller than that of the Pd foil (an effect due to particle size). Figure 2: In situ X-ray absorption studies. ( a , b ) XANES and EXAFS k -space spectra ( k 2 -weighted) from Au L3, and ( c , d ) from Pd K edges from the Pd 9 Au 1 nanoparticles measured in 1 M HClO 4 at a potential of 0.41 V (red lines), together with those from reference foils (blue lines). 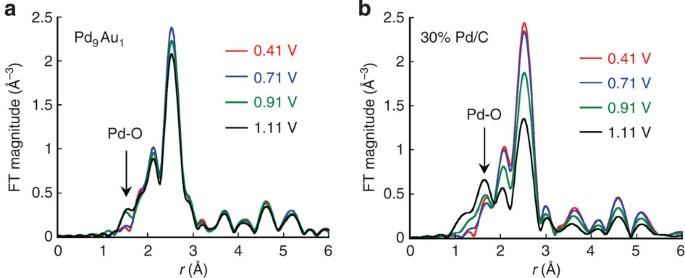Figure 3: Fourier-transformed EXAFS spectra. (a) Pd K edge from carbon-supported Pd9Au1alloy nanoparticles and (b) Pd K edge from Pd nanoparticles (30 wt%) in 1 M HClO4with different applied potentials. Full size image Figure 3 shows the findings from in situ EXAFS studies of Pd 9 Au 1 /C and Pd/C nanoparticles measured at different potentials (0.41–1.12 V). The peak around 1.6 Å in the figures reflects the formation of Pd oxide. Clearly, Pd 9 Au 1 /C has much lower potential dependence than does Pd/C, and Pd oxidation/dissolution in acid media is inhibited considerably by alloying Pd with a small concentration of Au (10 at%). One of the origins is likely to be the electronic effect from the alloying element of Au as we discussed above. Figure 3: Fourier-transformed EXAFS spectra. ( a ) Pd K edge from carbon-supported Pd 9 Au 1 alloy nanoparticles and ( b ) Pd K edge from Pd nanoparticles (30 wt%) in 1 M HClO 4 with different applied potentials. Full size image Supplementary Figure S3 plots the first shell-fitting results for the Pd 9 Au 1 nanoparticles at a potential of 0.41 V. There is good agreement between the fits and the original spectra; the results of coordination numbers are summarized in Table 1 . ( Supplementary Table S1 lists the bond lengths and passive electron reduction factors.) For an A–B binary solid–solution (random) alloy, the ratio (relative to the A atom) of the coordination number N A−A to N A−B is equal to the mole fraction ratio x A /x B of the elements in the bulk [14] , that is, N A−A / N A−B = x A /x B . The statistical distribution of the two elements is characterized by equal sums of coordination numbers of one metal to that of the other, that is, N A−M = N B−M . We obtained the ratios of the coordination numbers, N Au−Au / N Au−Pd =0.28 and N Pd−Pd / N Pd−Au =10.2, that is, in reasonably good agreement with the mole fraction ratios, x Au / x Pd =0.16 and x Pd / x Au =9.0, each within the range of their experimental errors. Furthermore, the sum of coordination numbers for Pd ( N Pd−Pd + N Pd−Au ) is 10.1, which agrees well with that of Au ( N Au−Au + N Au−Pd ) at 10.4, indicating a homogeneous distribution of Pd and Au atoms in the particles without any preferential accumulation of one metal around the other. The EXAFS analysis demonstrates the formation of homogeneous PdAu alloy nanoparticles. We note that the PdAu nanoparticles in our previous study [6] were not as homogeneous as the present ones, and we believe that the higher homogeneity may impart the better stability as discussed below. Table 1 Coordination numbers determined by the EXAFS experiment. 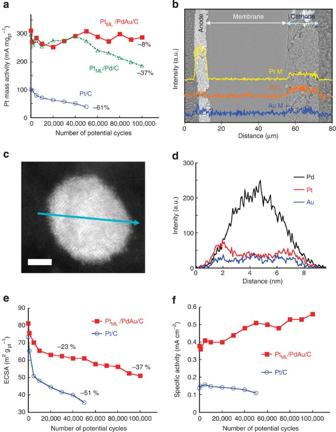Figure 4: Fuel cell stability test with potential cycles between 0.6 and 1.0 V (square wave) with a 10 s dwell time at 80 °C. (a) The Pt mass activity of the PtML/Pd9Au1/C electrocatalyst for the ORR at 0.9 V plotted as a function of the number of potential cycles during fuel cell testing. The results with PtML/Pd/C6and Pt/C catalysts are shown for comparison. Absolute pressure for H2/O2=150 kPa. Relative humidity=100%. (b) Scanning electron microscope picture of cross-section of the MEA with the concentration profiles of Pt, Pd and Au after 100,000 potential cycles. Pt loadings=0.105 mg cm−2for PtML/Pd9Au1/C, 0.102 mg cm−2for Pt/C. (c) HAADF/STEM image of carbon-supported PtML/Pd9Au1nanoparticle after 100,000 cycle test at potentials between 0.6 and 1.0 V. Bar size, 2 nm. (d) Distribution of components in the PtML/Pd9Au1nanoparticle obtained by the line-scan analysis using EDS/STEM (along the blue arrow inc). (e) The ECSA of the PtML/Pd9Au1/C and Pt/C electrocatalysts as a function of number of potential cycles during fuel cell testing. (f) The specific activity of the PtML/Pd9Au1/C and Pt/C electrocatalysts for the ORR at 0.9 V plotted as a function of the number of potential cycles during fuel cell testing. Full size table Stability test between 0.6 and 1.0 V Figure 4a depicts our results from stability tests of the Pt ML /Pd 9 Au 1 /C electrocatalyst, plotting Pt mass activity as a function of the number of potential cycles. The accelerated fuel-cell stability test involved potential step cycling between 0.6 and 1.0 V (square wave), with a 10-s dwell time at 80 °C. The stability of the electrocatalyst was excellent. After 100,000 cycles, the Pt mass activity did not change much (the initial value was 310 mA mg −1 ); it decreased by only 8%. We should note that the Department of Energy (DOE)'s target for 30,000 potential cycles is a loss of 40% (ref. 15 ). In the figure, we compare the results of the stability tests of Pt ML /Pd/C [6] (green triangles) and Pt/C (blue circles) electrocatalysts. The Pt mass activity of the Pt ML /Pd/C electrocatalyst was almost comparable to that of the Pt ML /Pd 9 Au 1 /C electrocatalyst up to 40,000 cycles, but then it declined to 37% after 100,000 cycles; this finding demonstrates that adding a small amount of Au to Pd cores effectively enhances the catalyst's stability. The Pt mass activity of the Pt/C catalyst (100 mA mg −1 ) was about three times less than that of the Pt ML /Pd 9 Au 1 /C electrocatalyst, and had decreased by 61% after 50,000 potential cycles. At the same stage, the Pt mass activity of Pt ML /Pd 9 Au 1 /C catalyst exhibited eight-fold enhancement over that of Pt/C. We note that the mass activity of Pt/C obtained in the present study is lower than that of the best benchmark result from 46% Pt/C catalyst (160 mA mg −1 ) under similar membrane electrode assembly (MEA) test conditions [1] , [15] . The DOE's 2017 target is 440 mA mg −1 (ref. 15 ). The initial PGM (precious-group metal) mass activity of Pt ML /Pd 9 Au 1 /C catalyst is 110 mA mg PGM −1 , which is almost comparable to that of Pt/C, but it did not change much with potential cycles and thus is 2.5 times higher than that of Pt/C after 50,000 cycles. The ORR activities measured by rotating disk electrode measurements from the Pt/Pd 9 Au 1 /C electrocatalyst are detailed in Supplementary Fig. S9 . Figure 4: Fuel cell stability test with potential cycles between 0.6 and 1.0 V (square wave) with a 10 s dwell time at 80 °C. ( a ) The Pt mass activity of the Pt ML /Pd 9 Au 1 /C electrocatalyst for the ORR at 0.9 V plotted as a function of the number of potential cycles during fuel cell testing. The results with Pt ML /Pd/C 6 and Pt/C catalysts are shown for comparison. Absolute pressure for H 2 /O 2 =150 kPa. Relative humidity=100%. ( b ) Scanning electron microscope picture of cross-section of the MEA with the concentration profiles of Pt, Pd and Au after 100,000 potential cycles. Pt loadings=0.105 mg cm −2 for Pt ML /Pd 9 Au 1 /C, 0.102 mg cm −2 for Pt/C. ( c ) HAADF/STEM image of carbon-supported Pt ML /Pd 9 Au 1 nanoparticle after 100,000 cycle test at potentials between 0.6 and 1.0 V. Bar size, 2 nm. ( d ) Distribution of components in the Pt ML /Pd 9 Au 1 nanoparticle obtained by the line-scan analysis using EDS/STEM (along the blue arrow in c ). ( e ) The ECSA of the Pt ML /Pd 9 Au 1 /C and Pt/C electrocatalysts as a function of number of potential cycles during fuel cell testing. ( f ) The specific activity of the Pt ML /Pd 9 Au 1 /C and Pt/C electrocatalysts for the ORR at 0.9 V plotted as a function of the number of potential cycles during fuel cell testing. Full size image Figure 4b shows a scanning electron microscope picture of a cross-section MEA, in which we placed a Nafion membrane between a Pt/C anode (left) and a Pt ML /Pd 9 Au 1 /C cathode (right), with the concentration profiles of Pt, Pd and Au after the 100,000 potential cycles. In our previous communication on the stability of Pt ML /Pd/C and Pt ML /PdAu/C cathodes [6] , we noted the formation of a Pd 'band' in the membrane after 100,000 potential cycles. We rationalized that a considerable amount of Pd had dissolved in the Pt ML /Pd/C and Pt ML /PdAu/C catalysts; those dissolved Pd 2+ ions that diffused out of the cathode catalyst layer into the membrane were reduced by H 2 permeating from the anode and, thereafter, deposited in the membrane and on the anode. The results, in Fig. 4b , showed no such 'band' formation; the dissolution of Pd in the new Pt ML /Pd 9 Au 1 /C catalyst was impeded considerably under the potential cycle test. The core-shell structure remains fairly after the test, as shown in a STEM/EDS line-profile analysis ( Fig. 4d ) on a nanoparticle ( Fig. 4c ). Figure 4e illustrated the changes in electrochemical surface area (ECSA) of the Pt ML /Pd 9 Au 1 /C and Pt/C electrocatalysts. The ECSAs were determined by hydrogen adsorption/desorption regions observed in voltammetry curves measured during the cycle tests ( Supplementary Fig. S4 ). The loss in ECSA of the Pt ML /Pd 9 Au 1 /C after the 100,000 cycle test is 37%, also much superior to the DOE's target (≤40% at 30,000 cycles). The loss in ECSA is presumably caused by disappearance of small particles due to electrochemical Ostwald ripening [4] ; the notion is supported by the fact that the mean diameter of the nanoparticles after the 100,000 cycle test became larger (4.1 nm) than the initial value (3.8 nm; Supplementary Fig. S1a,b ). The specific activity of Pt ML /Pd 9 Au 1 /C catalyst as a function of the number of potential cycles, determined by the mass activity and ECSA, is presented in Fig. 4f . The initial specific activity is 0.38 mA cm −2 , which is 2.7 times higher than that of Pt/C also shown in the figure. An intriguing feature is that it gradually increased to, for example, 0.51 mA cm −2 at 50,000 potential cycles. Two plausible factors for the enhancement in specific activity are considered; one is a slight contraction in Pt monolayer due to gradual dissolution of Pd [6] , [16] , and the other is re-arranging the surface atoms into smoother and higher-coordinated surfaces [17] . Density functional theory calculations We undertook density functional theory (DFT) calculations to elucidate the observed enhancement of the stability of the Pt ML /Pd 9 Au 1 /C electrocatalyst compared with that of Pt ML /Pd/C. To simulate the Pt monolayer electrocatalysts, we constructed sphere-like nanoparticle models of ~1.7 nm, based on a truncated octahedron ( Fig. 5 ). Our previous studies [16] , [18] demonstrated the success of the ~1.7 nm nanoparticle model to interpret the experimental trends in electrocatalytic activities. We first examined two Pd 9 Au 1 core models with 71 Pd and 8 Au atoms ( Supplementary Fig. S5 ). Model I was constructed by randomly substituting 25.0% of Au atoms for Pd atoms inside Pd 9 Au 1 and 75.0% of Au atoms on its surface (two and six atoms, respectively), whereas Model II was generated by substituting for Pd atoms only inside Pd 9 Au. Model I aims to simulate the well-mixed PdAu alloy, whereas Model II is considered as an extreme case. Here we did not consider the case of all the Au atoms in the shell according to our experimental observations ( Fig. 1 ). Our DFT calculations found that Model I is more stable than Model II by 2.78 eV. Accordingly, Model I was used to calculate the stability of Pt ML /Pd 9 Au 1 , by depositing Pt atoms on the surface as shown in Fig. 5 . To interpret the measured enhancement in stability, we examined the segregation of Au atoms (or the anti-segregation of Pd atoms) from the core (Pd 9 Au 1 ). It is known that owing to the imperfection of the Pt monolayer, Pt defective sites (Pt vacancies in this case) would be available ( Supplementary Fig. S6 ), which would lower the stability of the electrocatalysts. Therefore, before proceeding with our assessments of segregation, we compared the stability of defective sites using a 1.7 nm Pt nanoparticle. As compiled in Supplementary Table S2 , defects are likely to exist at the sites near or at the vertex ( D 2 or D 3 , respectively). Thus, we only simulated segregation by examining the diffusion of Au or Pd atoms from the core to the defective vertex sites on the surface ( Supplementary Fig. S6 ). As compiled in Supplementary Table S3 , the movement of Au from the core to the defective site ( Fig. 5a ) gains much more energy than that of Pd ( Fig. 5b ; −0.50 eV versus −0.14 eV, respectively), whereas the Pd segregation of Pt ML /Pd exhibits a similar energy gain compared with that of Pt ML /Pd 9 Au 1 (−0.16 eV versus −0.14 eV, respectively). Thus, our calculations clearly manifest that Au atoms preferentially remain on the surface by the segregation process; this will mend the defective sites on the Pt monolayers and, thus, markedly inhibit the Pd and Pt dissolution. Recent observations that preferential replacement of Au atoms takes place at the vertex or corner sites on Pd nanoparticle surfaces (1.8 nm diameter) [19] may also support our results. Accordingly, the stability of Pt ML /Pd 9 Au 1 /C under fuel-cell conditions may be augmented through the inhibition of Pd dissolution. 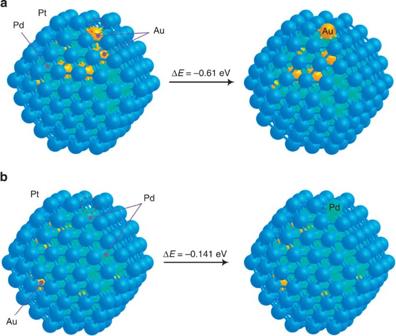Figure 5: DFT calculations to investigate the segregation effect. Geometrical illustrations depicting the segregation of (a) Au atoms and (b) Pd atoms from the core to the defective site in the Pt monolayer (Model I) for DFT calculations. The negative value indicates a more stable state. The relative energies are averaged ones as shown inSupplementary Table S3. Dashed circles are defective sites. Pt, Pd and Au atoms are in blue, sky blue and orange colours, respectively. Figure 5: DFT calculations to investigate the segregation effect. Geometrical illustrations depicting the segregation of ( a ) Au atoms and ( b ) Pd atoms from the core to the defective site in the Pt monolayer (Model I) for DFT calculations. The negative value indicates a more stable state. The relative energies are averaged ones as shown in Supplementary Table S3 . Dashed circles are defective sites. Pt, Pd and Au atoms are in blue, sky blue and orange colours, respectively. Full size image Stability test between 0.6 and 1.4 V The upper limit of potential range, that is, 1.0 V, was chosen from the stability test protocols specified by the DOE [15] . However, the higher potentials (≥ 1.4 V) would be applied to cathodes for automotive applications wherein frequent start/stop cycling is expected; this phenomenon, caused by the partial coverage of hydrogen and oxygen in the anode, would be the most hazardous one in PEMFC operations [20] , [21] . Tolerance under such high potentials is the key requirement for practical cathodes. 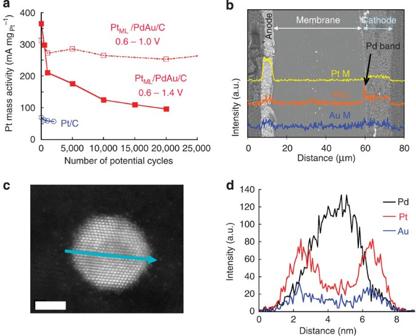Figure 6: Fuel cell stability test with potential cycles between 0.6 and 1.4 V (square wave) with a 10 s dwell time at 80 °C. (a) The Pt mass activity of the PtML/Pd9Au1/C electrocatalyst for the ORR at 0.9 V as a function of number of potential cycles during fuel-cell testing. The result with a Pt/C catalyst is shown for comparison. Absolute pressure for H2/O2=150 kPa. Relative humidity=100%. (b) Scanning electron microscope picture of cross-section of the MEA and the concentration profiles of Pt, Pd and Au after 20,000 potential cycles. Pt loadings in the cathodes: 0.105 mg cm−2for PtML/Pd9Au1/C, 0.102 mg cm−2for Pt/C. (c) HAADF/STEM image of carbon-supported PtML/Pd9Au1nanoparticle after 20,000 cycle test at potentials between 0.6 and 1.4 V. Bar size, 2 nm. (d) Distribution of components in the PtML/Pd9Au1nanoparticle obtained by the line-scan analysis using EDS/STEM (along the blue arrow inc). Figure 6a shows the Pt mass activity of the Pt ML /Pd 9 Au 1 /C electrocatalyst as a function of the number of potential cycles at potentials between 0.6 and 1.4 V. The activity decays sharply by 1,000 cycles, but then decreases slowly toward a value of ca 100 mA mg Pt −1 at 20,000 cycles. Even though this value is about 40% of that observed under the 0.6–1.0 V cycle test at 20,000 cycles (the dotted red curve in the figure), the Pt ML /Pd 9 Au 1 /C electrocatalyst undoubtedly is durable under the harshest condition in comparison with the plot from a Pt/C catalyst also shown in the same graph (blue circles). The activity of the Pt/C catalyst declines immediately after the cycle test; the ECSA by then showed an 81% loss compared with the initial area at 2,000 cycles ( Supplementary Fig. S7 ). The test of the Pt/C catalyst was terminated, as its activity was almost lost after 2,000 cycles; we found that Pt was significantly depleted in the cathode layer due to its dissolution. Figure 6: Fuel cell stability test with potential cycles between 0.6 and 1.4 V (square wave) with a 10 s dwell time at 80 °C. ( a ) The Pt mass activity of the Pt ML /Pd 9 Au 1 /C electrocatalyst for the ORR at 0.9 V as a function of number of potential cycles during fuel-cell testing. The result with a Pt/C catalyst is shown for comparison. Absolute pressure for H 2 /O 2 =150 kPa. Relative humidity=100%. ( b ) Scanning electron microscope picture of cross-section of the MEA and the concentration profiles of Pt, Pd and Au after 20,000 potential cycles. Pt loadings in the cathodes: 0.105 mg cm −2 for Pt ML /Pd 9 Au 1 /C, 0.102 mg cm −2 for Pt/C. ( c ) HAADF/STEM image of carbon-supported Pt ML /Pd 9 Au 1 nanoparticle after 20,000 cycle test at potentials between 0.6 and 1.4 V. Bar size, 2 nm. ( d ) Distribution of components in the Pt ML /Pd 9 Au 1 nanoparticle obtained by the line-scan analysis using EDS/STEM (along the blue arrow in c ). Full size image Figure 6b displays a scanning electron microscope picture of the cross-section of the MEA together with the EDS distribution of Pt, Au and Pd components after the 20,000 cycle test between 0.6 and 1.4 V. Potential cycling dissolved Pd in the cathode layer. A thin Pd-enriched band is seen at the interface between the membrane and cathode layer, viz. , a consequence of Pd dissolution and the reduction of Pd 2+ at the interface. An important observation here is that both Pt and Au in the cathode compartment survived under our harshest test, so far up to 20,000 cycles, whereas most Pt in the Pt/C dissolved after only 2,000 cycles. We note that the test protocol involving 1.0–1.5 V cycle with a triangular waveform has been suggested to evaluate the durability of support materials [22] ; although we have not followed that protocol, we consider that the durability of our catalyst under 1.0–1.5 V cycles would be higher than that obtained under the present condition. Figure 6c,d depicts an HAADF image of a single nanoparticle of Pt ML /Pd 9 Au 1 /C after the 20,000 cycle test between 0.6 and 1.4 V, and the EDS distribution of Pt, Au and Pd along the scanned line as indicated in Fig. 6a . The core-shell structure is maintained even after this treatment. However, there are three marked differences compared with the results before the cycle test ( Fig. 1 ) and after the 0.6–1.0 V potential cycle test ( Fig. 4c,d ). First, the relative intensity of Pd in the core compared with those of Pt and Au decreased apparently due to the dissolution of Pd atoms. Second, the Pt shell appears to be thickened as indicated by the increase in signal intensity at both the end sides of the particle in the EDS line profile ( Fig. 6d ). Third, at both edges of the nanoparticle, the Au intensity is also higher than that at the centre; this might partially reflect poor separation between the Pt L and Au L peaks in EDS, but might also suggests that the shell comprises a Pt–Au alloy layer. To further investigate the compositional distributions of Pt, Pd and Au in the nanoparticles, we carried out elemental mapping using EDS coupled with STEM. 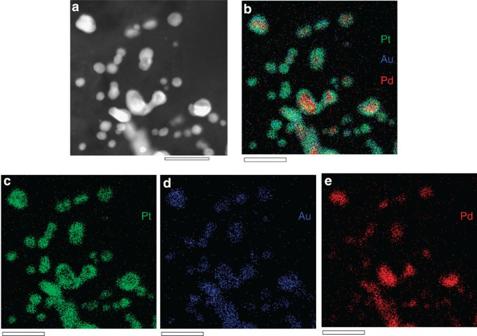Figure 7: Morphological and compositional observations after the cycle test between 0.6 and 1.4 V. (a) HAADF/STEM image of PtML/Pd9Au1nanoparticles and EDS elemental maps of (c) Pt, (d) Au and (e) Pd in the same area after the 20,000 cycles between 0.6 and 1.4 V. (b) EDS elemental map overlapping Pt (green), Au (blue) and Pd (red). Bar sizes, 20 nm. Figure 7a shows a HAADF/STEM image of Pt ML /Pd 9 Au 1 /C nanoparticles and EDS elemental mapping of Pt ( Fig. 7c ), Au ( Fig. 7d ) and Pd ( Fig. 7e ) in the same region after 20,000 cycles between 0.6 and 1.4 V. Figure 7b is an image of the overlapping Pt, Au and Pd compositional distributions. The distribution areas of Pt and Au are similar to the sizes of the nanoparticles ( Fig. 7a ), whereas those of Pd on average are smaller, presumably because they may have been consumed under the harsh test conditions. The core-shell structure was well retained ( Fig. 7b ) after the 20,000-cycle test except for a couple of small nanoparticles, in which the distribution of Pd atoms is hardly seen. Figure 7: Morphological and compositional observations after the cycle test between 0.6 and 1.4 V. ( a ) HAADF/STEM image of Pt ML /Pd 9 Au 1 nanoparticles and EDS elemental maps of ( c ) Pt, ( d ) Au and ( e ) Pd in the same area after the 20,000 cycles between 0.6 and 1.4 V. ( b ) EDS elemental map overlapping Pt (green), Au (blue) and Pd (red). Bar sizes, 20 nm. Full size image Mechanisms for high durability Among three constituents of this catalyst, Pd is the most reactive metal with the lowest standard electrode potential: As shown in Fig. 3 , Pd oxidation/dissolution is markedly inhibited when Pd is alloyed with 10 at% of Au. Alloying Pd with Au causes a positive shift of the Pd oxidation potential. Fang et al . [23] also reported that Au in Pd-Au nanoparticles can impart oxidation resistance to Pd. The inhibition of Pd oxidation/dissolution definitely is one of the factors accounting for the improved stability of the Pt ML /Pd 9 Au 1 /C electrocatalyst, and likely is caused by the electronic effect of Au on Pd. Several researchers studied the electronic inference between two elements in the Pd–Au system [24] , [25] , [26] . Metallic Au has completely filled the d- orbitals, and thus does not exhibit an intense peak (the so-called white line) at the L3 edge, as indicated by the dotted blue curve from an Au foil in Fig. 2a . However, the Au L3 spectrum from the Pd 9 Au 1 nanoparticles reveals an enhanced intensity in the white line (designated by an arrow) compared with that from the Au reference foil ( Fig. 2a ). The increase plausibly reflects a rise in the number of holes in d -band, as a result of the d -electron donation to Pd. On the other hand, the Pd K edge spectrum from the Pd 9 Au 1 nanoparticles exhibited a decrease in its peak intensity (designated by an arrow) compared with that from a Pd foil ( Fig. 2c ). Even though the primary transition for the Pd K edge spectrum is 1 s →5 p , the final state often may have hybridization (mixing) with other orbitals, and the Pd K adsorption edge is known to reflect a change in d -band density due to the extent of 4 d –5 p hybridization [27] , [28] , [29] . The observed lower intensity in K edge may be derived from a decrease in the number of d -holes, resulting from the filling of the d -band vacancies by electrons from Au. The decrease in strength of the Pd L3 white line by alloying with Au was also observed by others [30] , [31] . Such a reduction of the number of unoccupied d -electronic states may enhance the corrosion resistance of Pd, although detailed studies are necessary to establish an exact mechanism for any relationship between them. Pd atoms may dissolve through imperfection sites (vacancies) in Pt monolayers. The DFT calculation indicates that Au atoms segregate preferentially at defect sites in Pt monolayers; if Au atoms mend the defective sites, Pd dissolution from the cores will be effectively suppressed. This 'healing' effect by Au atoms is another factor for the improved stability. The segregated Au atoms on the surfaces also are beneficial in bettering the durability of the Pt monolayers. We demonstrated the stabilization of Pt nanoparticles in the presence of Au clusters under potential cycling conditions [32] . The Au clusters may be deposited preferentially at low-coordinated sites, such as defects and edges on the nanoparticles, to minimize the total free surface energy; the Au-clusters may block the initiation of Pt oxidation/dissolution and thereby stabilize the Pt surfaces. Even if the upper limit of the potential cycle rises to 1.4 V, Au appears to be immune from dissolution due to its high-standard electrode potential; however, the dissolution of Pd is unavoidable. One might have considered that Pt monolayers also would undergo profound dissolution under such harsh test conditions; this was not observed. It may well be that the Pd dissolution will prevent the cathode potential from reaching high values at which Pt dissolution easily takes place. In other words, Pd may exert a certain degree of cathodic protection on Pt [6] . As the Pd dissolution from the cores proceeds, the nanoparticles shrink gradually and the Pt monolayers collapse inward, which engenders a Pt bi-/multilayer formation as well as the formation of a hollow structure. The mean diameter of the nanoparticles after the 20,000-cycle test (0.6–1.4 V) was 3.6 nm, which is slightly smaller than the initial diameter, and that after the 100,000-cycle test between 0.6 and 1.0 V ( Supplementary Fig. S1 ). We argued earlier that the formation of a hollow structure might induce a slight contraction in Pt bonds and thereby enhance ORR activity [6] , [16] . Such a mechanism may be operative in the present system. Meanwhile, repetitive potential cycling induces the thicker Pt (and partially PtAu alloy shells) that may impede the diffusion of Pd atoms from the cores to the surfaces, thereby retarding the Pd dissolution rate. STEM studies on the cathode after 0.6–1.4 V cycle test revealed formation of smooth (111) and facets (100) on the surfaces of many nanoparticles ( Supplementary Fig. S8 ). Low-coordination sites are more prone to oxidation and dissolution [33] , [34] , [17] ; the potential cycling re-arranges the surface atoms (including the healing process of surface defects by Au atoms mentioned above), and the resulting smooth, high-coordinated surfaces may further increase the stability of this electrocatalyst [17] . We report a new class of highly durable and active electrocatalysts that comprise Pt monolayers on Pd–Au alloy nanoparticles. In fuel-cell stability tests, this ultra-low Pt content electrocatalyst showed a little degradation in activity during 100,000 cycles between potentials 0.6 and 1.0 V. No significant losses in metal constituents in the cathode electrocatalyst were observed. Furthermore, under more severe test conditions with a potential range of 0.6–1.4 V, there were no considerable losses of Pt and Au, although marked dissolution of Pd from the nanoparticles cores was observed. The experimental data coupled with theoretical analyses demonstrated that the Pt ML /Pd 9 Au 1 /C electrocatalyst is highly tolerant and promising for the automotive application of fuel cells. Catalyst synthesis Pd 9 Au 1 alloy nanoparticles (the mole ratio of Pd to Au is 9 to 1) were synthesized using wet impregnation of carbon particles (acetylene black) by Pd and Au chlorides, and chemical reduction by formic acid. We deposited Pt monolayers on PdAu nanoparticle surfaces using the galvanic displacement of a Cu monolayer by dissolved K 2 PtCl 4 (refs 8 , 35 , 36 ). A Cu monolayer was obtained by underpotential deposition of a Cu monolayer on the reduced surfaces of the Pd 9 Au 1 nanoparticles. The procedure of 2 g synthesis was described elsewhere [37] . Recently, the quantity of one batch was increased to 200 g. The total metal loading of the Pt ML /Pd 9 Au 1 /C is 40 wt%. STEM/EDS measurements were carried out using a JEM 2100F microscope. The mean diameter of the nanoparticles was determined as 3.8±1.2 nm ( Supplementary Fig. S1 ). MEA test A potential programme was applied to the cell comprising the MEA using H 2 at the anode (counter electrode) and N 2 at the cathode (working electrode) at 150 kPa absolute pressure and 100% relative humidity at 80 °C. We employed single cells with a surface area of 25 cm 2 and a Nafion NRE211CS membrane. Two different accelerated stability tests were carried out; one involved potential step cycling between 0.6 and 1.0 V (square wave), whereas the other was applied from 0.6 to 1.4 V. For both, the dwell time for each potential was 10 s. O 2 was injected in the cathode at 150 kPa absolute pressure and polarization curves were obtained with 100% relative humidity at 80 °C. In situ XAS XAS measurements using an electrochemical cell were undertaken at BNL's National Synchrotron Light Source at the X19A beamline. The Pd 9 Au 1 sample (working electrode), a proton exchange membrane (Nafion 117, DuPont Chemical Co., DE) and a Pt thin foil (counter electrode) were sandwiched and clamped tightly by the two acrylic plastic bodies. Each plastic body has an X-ray window. The electrolyte was 1 M HClO 4 and an Ag/AgCl leak-free electrode was used as a reference electrode. All potentials in this paper are quoted with respect to the reversible hydrogen electrode. Details of the electrochemical cell, which is a modified version of that described in ref. 38 , are given elsewhere [37] . The data acquired by both the electrochemical and thermal cells were processed and analysed by Athena and Artemis software [39] . Computational methods We carried out periodic DFT calculations using the Vienna ab initio simulation package [40] with projector-augmented wave [41] potentials and the revised Perdew–Burke–Ernzerhof exchange-correlation functional [42] . All calculations were carried out with a 400-eV kinetic energy cutoff value for a plane wave basis set using only the Γ -point for k -sampling. Spin-polarization calculations were used. Similar to our previous studies [16] , [18] , we employed sphere-like nanoparticle models with ~1.7 nm in diameter to simulate the core-shell nanoparticles (Pt ML /Pd and Pt ML /Pd 9 Au 1 ). In addition, for the subcore Pd 9 Au 1 simulations, two types of nanoparticle models with ~1.2 nm in diameter were generated with 71 Pd and 8 Au atoms. As shown in Supplementary Fig. S5 , in Model I, Au atoms are distributed over the shell and core of the particle, whereas in Model II they are located only in the core. In this study, all atoms were fully optimized. For defective structures of the Pt nanoparticle, each relative energy was calculated according to E rel = E [defective Pt NP]+ E [one Pt atom]− E [perfect Pt NP], where E represents the electronic energies of a defective Pt nanoparticle, one Pt atom calculated from bulk Pt and a perfect Pt nanoparticle. How to cite this article: Sasaki, K. et al . Highly stable Pt monolayer on PdAu nanoparticle electrocatalysts for the oxygen reduction reaction. Nat. Commun. 3:1115 doi: 10.1038/ncomms2124 (2012).